Reply to ‘Are atrial human pluripotent stem cell-derived cardiomyocytes ready to identify drugs that beat atrial fibrillation?’ 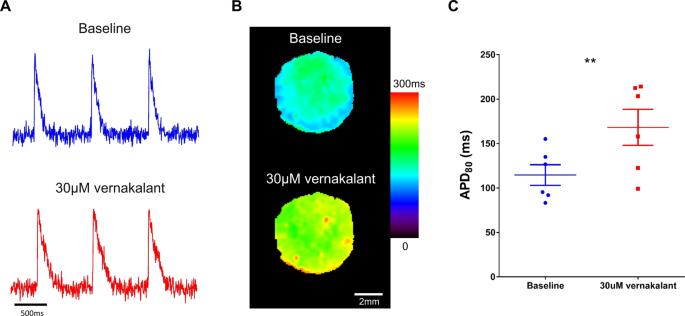Fig. 1: Effect of vernakalant on APD in hiPSC-derived atrial cell sheets. AExample of optical action potentials acquired from the two-dimensional hiPSC-derived atrial cell sheets at baseline (top) and following treatment with 30 µM vernakalant (bottom). Notice the atrial-like triangular-shaped optical action potential morphologies and the longer APD after the drug treatment.BAPD80color-coded maps depicting APD80values at each pixel of the atrial cell sheets at baseline (top) and following vernakalant treatment (bottom).CSummary of mean APD80values at baseline and upon administration of 30 µM vernakalant. Note the significant (**P= 0.0074, two-sided pairedttest,n= 6) APD80prolongation (from 115 ± 12 to 168 ± 20 ms) following the drug treatment. Source data is provided as aSource datafile. Generation and mapping of hiPSC-derived atrial tissues A hiPSC-derived atrial cardiomyocyte cell sheet model was prepared, as previously described [8] , [9] . Briefly, differentiated hiPSC atrial cells were seeded as dense 20 µl droplets containing ~700,000 cells on Matrigel-coated 35 mm plastic dishes. The resulting atrial cell sheets were cultured in 2 ml RPMI/B27 medium. At days 5–10, specimens were loaded with the voltage-sensitive dye FlouVolt and studied using an EM-CCD-based optical mapping system. Statistical analysis GraphPad Prism6 was used for statistical comparisons. Continuous variables are expressed as mean ± SEM. Paired t test was used to compare the effects of Vernakalant on the hiPSC-derived atrial cell sheets (Fig. 1 ) and on the ventricular EHTs (reanalysis of the data in Goldfract et al. [1] ). P < 0.05 was considered statistically significant. Reporting summary Further information on research design is available in the Nature Research Reporting Summary linked to this article.